Estimating the effective density of engineered nanomaterials forin vitrodosimetry The need for accurate in vitro dosimetry remains a major obstacle to the development of cost-effective toxicological screening methods for engineered nanomaterials. An important key to accurate in vitro dosimetry is the characterization of sedimentation and diffusion rates of nanoparticles suspended in culture media, which largely depend upon the effective density and diameter of formed agglomerates in suspension. Here we present a rapid and inexpensive method for accurately measuring the effective density of nano-agglomerates in suspension. This novel method is based on the volume of the pellet obtained by benchtop centrifugation of nanomaterial suspensions in a packed cell volume tube, and is validated against gold-standard analytical ultracentrifugation data. This simple and cost-effective method allows nanotoxicologists to correctly model nanoparticle transport, and thus attain accurate dosimetry in cell culture systems, which will greatly advance the development of reliable and efficient methods for toxicological testing and investigation of nano–bio interactions in vitro . The unique physical and chemical properties exhibited by engineered nanomaterials (ENMs), which are distinct from those of their micron-sized counterparts, and which endow them with exceptional performance in consumer products, may also be responsible for unique biological effects that can render them unsafe for humans and for the environment [1] , [2] , [3] . Efficient and cost-effective toxicological testing is therefore required to keep apace of the rapidly growing array of ENMs entering the consumer market [1] , [4] , and to enable studies that will provide a critical understanding of the relationships between the physicochemical properties of ENMs, including size, morphology, surface chemistry and crystallinity, and their biological effects. Given the high cost of animal testing, there is a pressing need for reliable high-throughput in vitro screening methods [1] , [4] , [5] , [6] . To date, however, despite the impressive progress made in developing high-throughput in vitro assays, the results have too often conflicted with those of animal studies [4] , [5] , [6] , [7] , [8] , [9] , [10] , and so have not earned widespread acceptance. Although differences between the two systems, particularly the interaction between multiple cell types and organismic processes operating in in vivo systems, which are absent in in vitro systems, may account for much of this disparity, it is likely that inaccurate characterization of in vitro dose, particularly failure to account for particle transformation and kinetics and their effect on mass transport of ENMs within cell culture systems, has contributed substantially to this problem [11] , [12] , [13] , [14] . In a typical cytotoxicity study, ENMs are suspended in media for application to cells in culture, and dose is reported as either the total particle mass, particle number, particle surface area or particle volume per unit volume of liquid media (concentration), or per unit sedimentation surface (surface area of the well [13] , [15] , [16] ). More recently, attention has been drawn to the mass transport (sedimentation and/or diffusion) of particles in suspension, which proceeds at a rate governed by the mass transport properties (sedimentation and diffusion coefficients) of the formed agglomerates in suspension [13] , [16] , [17] . These suspended forms are in most cases agglomerates consisting of multiple primary ENM particles as well as trapped suspension fluid and associated proteins as depicted in Fig. 1a . The fate and transport of the formed agglomerates in suspension determine the effective dose delivered to cells [11] , [12] , [13] , [14] . Accurate dosimetry therefore requires accurate characterization of agglomerate properties, particularly their effective diameter and density, which, along with the density and viscosity of the suspending fluid, determine mass transport phenomena (See Supplementary Note 1 , Supplementary equations (1–11) for detailed treatment of mass transport phenomena). Within the typical size range of the agglomerated forms found in in vitro experimental nanotoxicology systems (~100–300 nm), although diffusion does occur, transport is dominated by sedimentation, and it is therefore particularly important to characterize the properties that govern that process, specifically diameter and effective density [12] , [13] , [14] . Whereas the effective diameter (applicable to transport), denoted as the hydrodynamic diameter, d H , is readily measured by contemporary analytical methods such as dynamic light scattering (DLS), and is sufficient for modelling the diffusion component of transport, determination of agglomerate density, necessary for modelling sedimentation, presents a greater challenge. The effective density of nano-agglomerates in liquid suspension refers to the density of the agglomerate unit, which includes both particles and media components, as opposed to the density of the primary particle, which is simply the density of the raw ENM material. For flame-generated fractal nanomaterials, particle interactions in cell culture media typically used for in vitro toxicity assays may lead to the formation of agglomerates with media and proteins trapped within its empty spaces ( Fig. 1a ). Because the entrapped media and proteins often have considerably lower density than the primary particles, the effective density of the agglomerate unit can be significantly lower than that of the raw material [13] , [16] . The Sterling equation, based on a fractal model of agglomerate structure, has been used to obtain rough estimates of agglomerate effective density [18] ( Supplementary Note 2 ; Supplementary equations (12) and (13) ). This equation, however, requires a theoretical fractal dimension (DF) value for the agglomerated ENM, which can be neither measured nor verified, and the practical validity of this approach thus remains unproved. Alternatively, the sedimentation coefficient of a suspended ENM can be measured directly by analytical ultracentrifugation (AUC) [19] , [20] , thereby eliminating the need to explicitly determine effective density. Although the combination of DLS and AUC results may provide accurate measurement of ENM-effective density, AUC requires relatively expensive equipment that is not readily available to many nanotoxicology labs, and is moreover limited by a low throughput of at best several samples per hour, which would render the task of characterizing the thousands of ENMs that await testing an impractically costly and time-consuming one. 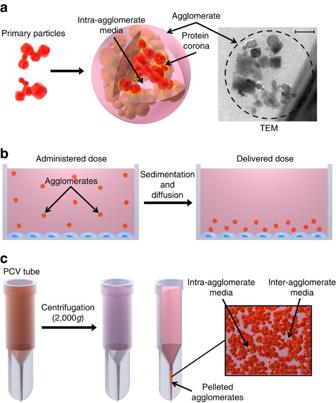Figure 1: Agglomeration of ENMs, transport in culture and volumetric centrifugation. (a) ENM primary particles suspended in cell culture media exist as agglomerates consisting of multiple primary particles, which may be enveloped by a corona of proteins from the media, and media trapped between primary particles (intra-agglomerate media). The TEM image of CeO2agglomerates suspended in RPMI/10% FBS was acquired with a JEOL 2100 microscope fitted with a Poseidon 500. Scale bar represents 50 nm. (b) ENM agglomerates within suspensions applied to cells settle towards the cells over time as a result of mass transport (sedimentation and diffusion). The initial administered dose is the concentration of ENM in the initially homogeneous suspension. As transport progresses, agglomerates are concentrated near or deposited onto the cells. The mass of ENM deposited per area is the delivered dose. (c) In volumetric centrifugation, a sample of ENM suspension is centrifuged in a PCV tube to produce a pellet, the volume of which can be measured and used to estimate the effective density of the ENM in suspension. The pellets contain both packed agglomerates and the media remaining between them (inter-agglomerate media). We refer to fraction of the pellet volume occupied by agglomerates as the stacking factor (SF). Figure 1: Agglomeration of ENMs, transport in culture and volumetric centrifugation. ( a ) ENM primary particles suspended in cell culture media exist as agglomerates consisting of multiple primary particles, which may be enveloped by a corona of proteins from the media, and media trapped between primary particles (intra-agglomerate media). The TEM image of CeO 2 agglomerates suspended in RPMI/10% FBS was acquired with a JEOL 2100 microscope fitted with a Poseidon 500. Scale bar represents 50 nm. ( b ) ENM agglomerates within suspensions applied to cells settle towards the cells over time as a result of mass transport (sedimentation and diffusion). The initial administered dose is the concentration of ENM in the initially homogeneous suspension. As transport progresses, agglomerates are concentrated near or deposited onto the cells. The mass of ENM deposited per area is the delivered dose. ( c ) In volumetric centrifugation, a sample of ENM suspension is centrifuged in a PCV tube to produce a pellet, the volume of which can be measured and used to estimate the effective density of the ENM in suspension. The pellets contain both packed agglomerates and the media remaining between them (inter-agglomerate media). We refer to fraction of the pellet volume occupied by agglomerates as the stacking factor ( SF ). Full size image We conceived a simple, low-cost, high-throughput method for estimating effective density based on the volume of the pellet obtained by low speed, benchtop centrifugation of an ENM suspension in a packed cell volume (PCV) tube. In this report, we present our rationale for and results from this method, which we refer to as the volumetric centrifugation method (VCM). Our findings demonstrate close agreement between our VCM approach and gold-standard AUC data for various classes of materials including flame-generated fractal ENM agglomerates as well as non-agglomerating nanospheres. We also demonstrate that the effective density estimated by this method can be used to accurately determine the rate of ENM agglomerate deposition and thus delivered dose of ENM in an in vitro system. Numerical estimates of delivered dose are validated for various materials using a novel neutron-activated tracer particle system, highlighting the utility and accuracy of employing direct measurement of effective density via VCM to calculate the dose delivered to cells over time. This simple and cost-effective method allows nanotoxicologists to correctly model nanoparticle transport, and thus attain accurate dosimetry in cell culture systems, which will greatly advance the development of reliable and efficient methods for toxicological testing and investigation of nano–bio interactions in vitro . Volumetric centrifugation method The PCV tube, originally designed and typically used for measuring biomass of cultured mammalian cells [21] , consists of a wide-bore sample loading upper chamber that tapers to a volumetric pellet-capturing capillary ( Fig. 1c ). In volumetric centrifugation, a sample of ENM suspension is centrifuged in a PCV tube to produce a pellet consisting of both packed agglomerates and the media remaining between them (inter-agglomerate media) ( Fig. 1c ). In the ideal case, assuming perfect stacking of ENM agglomerates with no intervening space, the total volume of agglomerate in a sample of ENM suspension, V agg , is simply the measured volume of the pellet collected by centrifugation, V pellet . Since the volume of ENM, V ENM , is readily derived from the known mass of ENM in suspension and the material density, the volume of the media trapped within agglomerates, V media , can be calculated as The effective density of the agglomerates, ρ EV , can then be calculated as a volume weighted average of ENM density, ρ ENM , and media density, ρ media , as However, in reality, the stacking of agglomerates is not perfect, and media remains interspersed between the stacked agglomerates (inter-agglomerate media, distinct from intra-agglomerate media, See Fig. 1c ). Thus, V agg comprises a fraction of the pellet, which we define as the stacking factor, SF : Substituting the right side of equation (3) for V agg inequations (1) and (2), replacing V ENM with the equivalent in terms of the ENM density, ρ ENM , and ENM mass, M ENM , and simplifying, yields For soluble materials, we must account for the portion of the original sample mass that is solubilized and which therefore does not contribute to the suspended agglomerate volume. This can be accomplished by subtracting the solubilized mass ( M ENMsol ), which can be measured, for example, by ICP-MS, from M ENM in equation (4): (See Supplementary Note 3 ; Supplementary equations (14–22) for a full derivation of equations (4) and (5)). Failure to account for this loss of the solubilized portion of the mass from M ENM would result in overestimation of effective density for these materials. The value of SF depends on the efficiency of agglomerate stacking. In the case of uniform spheres, possible values for SF may range from 0.634 for random close stacking [22] , to the theoretical maximum of 0.74 for ordered stacking [23] . For the roughly spherical agglomerates typically observed with nano metal and metal oxide ENMs (see EM image, Fig. 1a ), we expect SF values to approximate the theoretical value for random close stacking (0.634), whereas for non-agglomerating spherical ENMs, we expect SF to approach the theoretical value for ordered stacking (0.74). These theoretical SF values can be verified from the sedimentation coefficients measured for representative ENMs of each type using AUC. Specifically, from the sedimentation coefficient, s , of an ENM in liquid suspension measured by AUC ( Supplementary Note 1 ; Supplementary equations (9) and (10) ), the agglomerate density can be expressed as where η is the viscosity of the suspending media. The stacking factor can then be obtained by equating ρ EV in equation (4), and ρ agg in equation (5) and solving for SF , to yield Stacking factor validation Stacking factors were calculated for representatives of two major classes of ENMs (agglomerating flame-generated metal oxides and non-agglomerating metal nanospheres) from sedimentation coefficients measured by AUC with structure-insensitive interference detection (see Methods). As examples of flame-generated metal oxide ENMs, which exhibit similar chain-like aggregated primary particle morphologies and form roughly spherical agglomerates ( Supplementary Fig. 1 ), and which we therefore assume have similar stacking efficiencies, we estimated SF for CeO 2 ( d H =179 nm) and SiO 2 ( d H =135 nm). As a representative of a uniform spherical, non-agglomerating metal ENMs, we estimated SF for gold nanospheres suspended in DI H 2 O ( d H =29 nm). Stacking factors for the CeO 2 , SiO 2 and gold nanospheres were estimated from AUC sedimentation coefficient profiles (provided in Supplementary Fig. 2 ) to be 0.610, 0.538 and 0.764, respectively. The SF value of 0.610 and 0.538 for flame-generated CeO 2 and SiO 2 particles are, as expected given their spherical agglomerate shape, close to the theoretical value of 0.634 for random stacking of uniform spheres, and the SF of 0.764 for gold nanospheres is very close to the theoretical value of 0.74 for ordered stacking of uniform spheres. Therefore, for the family of agglomerating metal and metal oxide ENMs, which comprises 90% by volume of ENMs in the market [24] , the theoretical SF value of 0.634 provides a reasonable approximation. Similarly, the theoretical SF value of 0.74 is a suitable estimate for non-agglomerating nanometals. The aptness of these approximations is further supported by the fact that small differences in SF result in even smaller differences in ρ EV . For example, using the theoretical rather than measured SF values to calculate ρ EV for CeO 2 and SiO 2 alters the result by only 1.2% in the case of CeO 2 (from 1.492 to 1.474 g cm −3 ) and by 1.7% in the case of SiO 2 (from 1.131 to 1.112 g cm −3 ). Further, replacing the estimated SF for CeO 2 with a value 50% larger than the measured SF (0.910) results in only an 11% change in calculated ρ EV , from 1.492 to 1.333 g cm −3 . It is thus clear that effective density is relatively insensitive even to considerable errors in SF , and that we can therefore confidently employ the theoretical values in our method. Effective densities of ENMs by VCM and Sterling equation Effective densities of several widely used ENMs were measured by VCM, and results were compared with densities obtained using the Sterling equation. ENMs studied included flame pyrolysis-generated metal oxides currently under investigation by the Organization for Economic Cooperation and Development [25] , as well as non-agglomerating, gold nanospheres developed for biomedical applications. ENM properties, including crystal size, specific surface area, morphology, hydrodynamic diameter and zeta potential in suspension, were characterized using contemporary analytical techniques, as described in methods. Additional ENM dispersion properties and representative transmission electron microscopy (TEM) images of ENMs are shown in Supplementary Table 1 and Supplementary Fig. 1 respectively. Suspensions of ENMs, stably dispersed in cell culture media using protocols developed and previously reported by the authors [16] , were centrifuged in PCV tubes for 1 h at 2,000 g . In order to ensure that all of the suspended ENM was contained within the pellet, we analysed supernatants, collected after centrifugation at various speeds, by inductively coupled plasma mass spectrometry (ICP-MS). 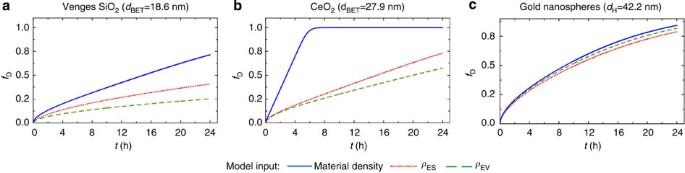Figure 2: Role of effective density in the rate of ENM deposition. Modelling of transport over time demonstrates the important role of ENM density in determining the rate of ENM deposition, indicated here byfD, the fraction of the administered dose (total mass of ENM in suspension) deposited at a given time. Assuming a density equal to that of the raw material (solid lines) results in an overestimation of deposition rate to a degree that depends upon the tendency of the ENM to form agglomerates that contain trapped media. Deposition rate curves are shown for three of the ENMs investigated suspended in cell culture media typically used forin vitronanotoxicology study (RPMI/10% FBS): (a) VENGES SiO2(dBET=18.6 nm). (b) CeO2(dBET=27.9 nm). (c) Gold nanospheres (dH=42.2 nm). The dotted and dashed lines represent deposition based on densities determined by volumetric centrifugation and the Sterling method, respectively. This analysis verified that negligible amounts of ENMs remained in suspension following centrifugation (See Supplementary Table 2 ). ENM-effective density, ρ EV , was estimated from measured pellet volume as described above using equation (4). The theoretical SF value for randomly stacked spheres (0.634) was used to calculate ρ EV for all metal oxide ENMs, and the theoretical SF value for ordered stacking of spheres (0.74) was used for the non-agglomerating gold particles (See Table 1 ). Table 1 ENM properties and effective densities by volumetric centrifugation and Sterling method. Full size table Effective densities estimated by VCM ( ρ EV ) and using the Sterling equation ( ρ ES ) are summarized in Table 1 . Whereas gold nanospheres exhibited a ρ EV value only slightly less than the density of elemental gold (17.73 versus 19.3 g cm −3 ), consistent with minimal agglomeration, all other ENMs exhibited ρ EV values closer to the density of the dispersion media (RPMI/10% fetal bovine serum (FBS), 1.0084, g cm −3 ) than to that of the raw ENM. This is a clear indication that ENMs formed agglomerates containing large amounts of trapped intra-agglomerate media (see Fig. 1a ). It is worth noting that since ρ EV values approach the density of the dispersion media as ENMs become more extensively agglomerated, that ρ EV also represents an indirect indicator of an ENM’s agglomeration potential (degree of agglomeration in suspension). In general, ρ EV for flame-generated metal oxide ENMs correlated with raw material density, which may suggest that agglomerates of these ENMs are composed of comparable relative proportions of particles and trapped media. Effective density also correlated with primary particle size among the three CeO 2 ENMs investigated ( ρ EV of 2.358, 1.625 and 1.474 g cm −3 for CeO 2 with d BET of 71.3, 27.9 and 5.4 nm, respectively). For many of the ENMs investigated ρ EV and ρ ES (estimated by the Sterling equation) were in reasonably close agreement. In those cases in which the results of the two methods did not agree, ρ ES was generally greater than ρ EV . This was most evident in the case of CeO 2 ( d BET =71.3 nm) for which the value of ρ ES was more than twice that of ρ EV . The small variation observed among triplicate measurements (<5% s.d., Table 1 ) for all materials examined suggests that the proposed method is both highly reproducible and robust. This is further demonstrated by the close agreement between our VCM results and those obtained via the gold-standard AUC method (AUC) ( Supplementary Fig. 2 ) for both a relatively high-density material (CeO 2 ), and a relatively low-density material (SiO 2 ), as well as for non-agglomerating gold nanospheres. However, it should be noted that slight variations in media formulation or dispersion protocol can result in differences in agglomeration state and thus effective density. For example ρ EV of CeO2 ( d BET =5.4 nm) is 1.473 g cm −3 in RPMI/10% FBS versus 1.374 g cm −3 in F12K/10% FBS. Dispersion protocol can also greatly influence agglomeration state, polydispersity and stability, and has been a source of much inconsistency in the past. Recently, however, a standardized protocol has emerged [16] , [25] , [26] , which was used in the present study, and has been proven to result in highly reproducible and stable suspensions [16] , [27] , [28] , [29] . Effective density stability over time All ENM suspensions in this study were prepared using a recently developed protocol that ensures sonication above the critical energy required to achieve small agglomerates that are stable in size over time (for 24–48 h (ref. 16 )). Other groups have also reported stable agglomerate sizes over 24–48 h using similar protocols for insoluble metal oxide ENMs [27] , [28] , [29] . In order to verify that the effective density of insoluble ENMs is stable over the time, we measured the effective density of a representative insoluble material following incubation in cell culture media for up to 24 h. CeO 2 ( d BET =27.9 nm) suspended in RPMI/10% FBS maintained a relatively stable effective density: ρ EV =1.474 g cm −3 immediately following dispersion, 1.440 g cm −3 at 4 h, and 1.442 g cm −3 at 24 h. These data confirm the relative stability of effective density over time for insoluble ENMs. For partially soluble materials, dynamic changes to agglomerate size and effective density over time must be accounted for in the fate and transport algorithm (for example, in vitro sedimentation diffusion dosimetry model, ISDD), in order to accurately estimate delivered dose. For these materials, equation (5), which accounts for the solubilized component, must be used to calculate effective density. For example, the VCM method was utilized to measure the effective density of ZnO ENMs ( d BET =63 nm) following 24-h incubation in cell culture media. To account for the effect of ion shedding on agglomerate density, we used the 35% dissolution reported for ZnO at 24 h (ref. 30 ) in equation (5). The effective density for this material decreased from 1.65 g cm −3 immediately following suspension to 1.37 g cm −3 after a 24-h incubation. These data suggest that dissolution not only reduces the mass of the particulate form, for which equation (5) provides the appropriate correction, but can also have a significant impact on agglomeration state and effective density. Thus, for partially soluble ENMs, accurate dosimetry would require comprehensive time-resolved dissolution as well as effective density measurements, in addition to a fate and transport model capable of employing such time-resolved dissolution and density data. Effect of ENM concentration and suspending media We performed additional experiments to assess the effect of initial ENM concentration and suspending media formulation on ρ EV measured by VCM. 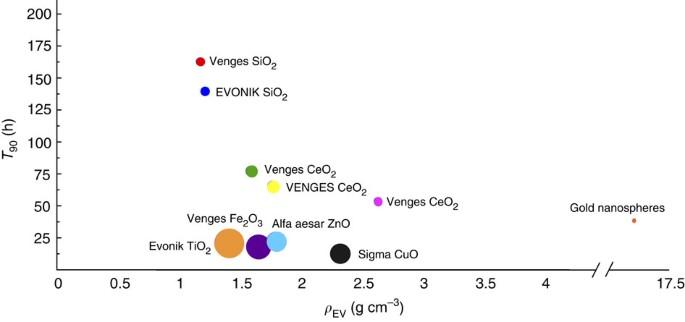Figure 3: Roles of agglomerate density and diameter in particle delivery to cells. Density and particle size both play important roles in determining the rate of ENM deposition. The combined effects of these two parameters results in a wide range, among the ENMs investigated, in the rate of deposition and consequently the time required for 90% of the ENM in suspension to be deposited, indicated here byT90. Effective density (ρEV) is represented along thexaxis. The diameter of the bubbles corresponding to each ENM represents and is relatively scaled to the agglomerate or hydrodynamic diameter (dH) of the ENM. Differences in ρ EV measured over a range of initial ENM concentrations typically used for nanotoxicity studies (50–250 μg cm −3 ) were negligible (≤7%, see Supplementary Table 3 ). 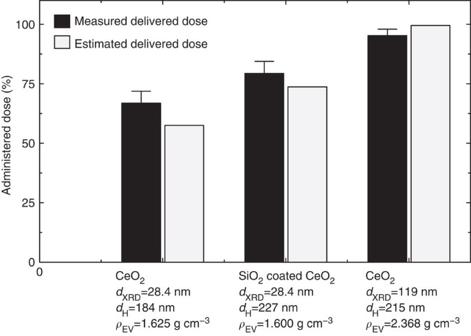Figure 4: Validation of VCM effective density and dosimetry approach. In order to validate the proposed dosimetry approach based on effective densities determined by VCM, suspensions of flame-generated and neutron-activated ENMs (CeO2(dXRD=28.4 nm), SiO2-coated CeO2(dXRD=28.4 nm) and CeO2(dXRD=119 nm) suspended in DMEM/5% FBS) were applied to transwell insert membranes with 3 μm pores. Following 24-h incubation, delivered dose was measured by gamma spectroscopy, defined as the sum of particles that deposited on or passed through the porous transwell insert membrane. Differences between delivered doses measured by the transwell approach and those estimated by particle transport modeling based on effective density calculated by VCM was <9% for all three materials tested. All experiments were done in triplicate. Error bars represent s.d. Differences among three media formulations tested (RPMI alone, RPMI+10% FBS and F12K+10% FBS) were somewhat larger (≤12%, see Supplementary Table 4 ), consistent with the dependence of agglomerate structure on media particle-specific properties [16] ( Supplementary Table 4 ). Stability of ENM agglomerates during centrifugation Although forces exerted on ENMs during low-speed centrifugation are exceedingly small (in the fN range), in order to rule out the possibility that agglomerate structures were altered by centrifugation, we performed atomic force microscopy experiments. Forces up to six orders of magnitude greater than those experienced during centrifugation were applied to agglomerates deposited onto a sample grid either prior to or following centrifugation (See Supplementary Methods ) and the deformation of agglomerates was assessed. The results of these experiments (See Supplementary Figs 3 and 4 ) revealed that forces experienced by agglomerates during low-speed centrifugation do not result in their deformation, and that agglomerates maintained their original architecture as expected. Further analysis of agglomerate stability is provided in the Supplementary Discussion . Role of effective density in ENM transport in vitro To examine the impact of effective density on ENM delivery to cells in vitro , we used the recently developed ISDD model to compute the fraction of administered ENM that would be deposited on cells over time, assuming a particle density of either the raw ENM material, ρ ENM , the VCM measured effective density, ρ EV , or the Sterling model effective density, ρ ES . Representative results, illustrated in Fig. 2 , demonstrate that the assignment of density substantially affects the rate of ENM deposition. In general, deposition calculated based on either ρ EV or ρ ES proceeds more slowly than that calculated based on ρ ENM . Moreover, with the exception of non-agglomerating gold nanospheres, for which all three densities, and accordingly all three corresponding deposition rates, are nearly identical, deposition at ρ EV proceeds more slowly than at ρ ES , as determined by the relatively lower densities estimated by the VCM approach. Figure 2: Role of effective density in the rate of ENM deposition. Modelling of transport over time demonstrates the important role of ENM density in determining the rate of ENM deposition, indicated here by f D , the fraction of the administered dose (total mass of ENM in suspension) deposited at a given time. Assuming a density equal to that of the raw material (solid lines) results in an overestimation of deposition rate to a degree that depends upon the tendency of the ENM to form agglomerates that contain trapped media. Deposition rate curves are shown for three of the ENMs investigated suspended in cell culture media typically used for in vitro nanotoxicology study (RPMI/10% FBS): ( a ) VENGES SiO 2 ( d BET =18.6 nm). ( b ) CeO 2 ( d BET =27.9 nm). ( c ) Gold nanospheres ( d H =42.2 nm). The dotted and dashed lines represent deposition based on densities determined by volumetric centrifugation and the Sterling method, respectively. Full size image These results illustrate the important contribution of density to sedimentation velocity ( Supplementary equation (9) ), and underscore the importance of the characterization of ENM transformations and agglomerate properties in calculating the dose delivered to cells in an in vitro system. The time required for 90% of administered ENM to be deposited, t 90, estimated from ISDD model outputs based on ρ EV and d H for all ENMs studied using previously described methods [16] , was also calculated and illustrated in Fig. 3 . These results further demonstrate the importance of effective density, along with agglomerate size, in determining the time required for ENM delivery, with ENMs having relatively greater values for both ρ EV and d H being deposited most rapidly and those with smaller values for both properties being deposited most slowly (for example, CuO, d H =310 nm, ρ EV =2.214 g cm −3 , t 90 =16 h versus VENGES SiO 2 , d H =135 nm, ρ EV =1.131 g cm −3 , t 90 =171 h). Figure 3: Roles of agglomerate density and diameter in particle delivery to cells. Density and particle size both play important roles in determining the rate of ENM deposition. The combined effects of these two parameters results in a wide range, among the ENMs investigated, in the rate of deposition and consequently the time required for 90% of the ENM in suspension to be deposited, indicated here by T 90 . Effective density ( ρ EV ) is represented along the x axis. The diameter of the bubbles corresponding to each ENM represents and is relatively scaled to the agglomerate or hydrodynamic diameter ( d H ) of the ENM. Full size image Effective density and delivered dose for soluble materials Because dissolution and agglomeration are dynamic processes, the portion of mass dissolved, and agglomerate size and density may vary over time for soluble materials. Thus for greatest accuracy M ENMsol and d H , and from these ρ EV , should be measured over the time of exposure. These time-resolved values should then be utilized by the transport simulation model (that is, ISDD) to accurately estimate delivered dose. We should also note that for soluble materials such as ZnO and CuO, the dosimetry data presented in Fig. 3 is limited by the fact that effective density measurements were obtained immediately following dispersion, and do not reflect dissolution during dispersion or the dynamic nature of agglomerate size and density due to dissolution over time. In light of this limitation, the data presented remain useful primarily for comparison of the material densities with the agglomerate effective densities (which are likely overestimated), and to highlight the impact of effective density on particle delivery to cells in vitro . In addition, for completion of dosimetry calculations, both the particulate and soluble components must be correctly identified and considered separately in order to properly assess the mechanistic effects of both ionic and particulate portions of the dose [31] , [32] . The ionic exposure component may be also reported as the dose of soluble ions per volume exposure media or per cm 2 sedimentation surface (surface area of the cell culture well). Experimental validation of VCM-derived delivered dosimetry In order to validate the proposed dosimetry approach based on effective densities determined by VCM, suspensions of three flame-generated and neutron-activated ENMs (CeO 2 ( d XRD =28.4 nm), CeO 2 ( d XRD =119 nm) or SiO 2 -coated CeO 2 ( d XRD =28.4 nm)) were applied to transwell insert membranes with 3 μm pores ( Supplementary Fig. 5 ). This is a well-established method for accurately tracking gamma emitting isotopes, in this case 141 Ce, with high sensitivity and correlates extremely well with total particle mass [33] . Following 24-h incubation, delivered dose was measured by gamma spectroscopy, defined as the sum of particles that deposited on or passed through membrane. Evaluation of membranes for particle loss (by adherence of particles to the membrane) confirmed that for all three materials tested more than 98% of particles passed freely through the membrane pores without adhering (data not shown). The results, summarized in Fig. 4 , reveal a close agreement (<9% difference) between the percent of administered dose measured in the basolateral compartments of the transwell system and the delivered doses based on effective densities measured by VCM. This is a clear validation of the proposed dosimetric approach for ENMs and indicates that the VCM method provides accurate measurements of effective density of the ENM agglomerates. Figure 4: Validation of VCM effective density and dosimetry approach. In order to validate the proposed dosimetry approach based on effective densities determined by VCM, suspensions of flame-generated and neutron-activated ENMs (CeO 2 ( d XRD =28.4 nm), SiO 2 -coated CeO 2 ( d XRD =28.4 nm) and CeO 2 ( d XRD =119 nm) suspended in DMEM/5% FBS) were applied to transwell insert membranes with 3 μm pores. Following 24-h incubation, delivered dose was measured by gamma spectroscopy, defined as the sum of particles that deposited on or passed through the porous transwell insert membrane. Differences between delivered doses measured by the transwell approach and those estimated by particle transport modeling based on effective density calculated by VCM was <9% for all three materials tested. All experiments were done in triplicate. Error bars represent s.d. Full size image It is also worth noting that the fate and transport numerical model used here (ISDD model) has been partially validated only for non-agglomerating, non-industrially relevant fluorescently labelled polystyrene spheres of various agglomerate diameter [13] , [34] and super paramagnetic iron oxide particles [13] . These results therefore provide the first validation for the ISDD model using industrially relevant ENMs. In Vitro Toxicity Characterization In order to evaluate the potential impact of effective density and particokinetics on in vitro toxicity assessment, we compared administered and delivered mass dose-responses for a representative ENM (CeO 2 , d BET =27.9 nm, ρ EV =1.625 g cm −3 ). Adherent human airway epithelial cells (Calu-3) were exposed for either 24, 48 or 72 h over a range of administered doses, mean delivered doses (averaged over time of exposure) were calculated by the VCM-ISDD model based on ρ EV and d H , and cytotoxicity was assessed by the WST-1 assay as described in methods. Supplementary Fig. 6 illustrates the substantial difference between administered and delivered dose-response curves for CeO 2 , which suggests that the administered dose (which assumes complete deposition of suspended material) substantially underestimates the toxicity of this material. For example, the maximum dose evaluated for the 24-h time point decreases from 31.6 μg cm −2 to 11.4 μg cm −2 when administered dose is converted to delivered dose. These results, though preliminary, highlight the potential importance of accurate measurement of effective density and particokinetics in in vitro dosimetry for nanotoxicology studies. In a separate meta-analysis of previously published cytotoxicity data for CoO and Co 3 O 4 nanoparticles [30] based on the LDH assay in BEAS-2B cells, dose-response curves generated using doses based on agglomerate size and effective density revealed a substantial change in relative hazard ranking of these materials compared with that based on administered dose-response curves. As depicted in Supplementary Fig. 7a , the dose-response curves based on administered dose values suggest that CoO is considerably more toxic than Co 3 O 4 , especially at administered doses of 5 μg and above. However, the VCM revealed that CoO has an effective density almost twice that of Co 3 O 4 (CoO, ρ EV =2.39 g cm −3 versus Co 3 O 4 ρ EV =1.37 g cm −3 ), and as a result the delivered dose of Co 3 O 4 was significantly lower than the delivered dose of CoO after a 24-h exposure. The resulting delivered dose-response curves ( Supplementary Fig. 7b ) suggest that Co 3 O 4 is nearly as cytotoxic as CoO on a delivered mass basis. Effect of polydispersity As a further validation of the proposed VCM approach, we assessed the possible error in dosimetry due to polydispersity of ENM agglomerate density ( Supplementary Fig. 8 ). Our results suggest that faster-settling and slower-settling agglomerates roughly balance, such that the total particle calculated by the ISDD model using average values for d H and ρ EV does not differ greatly from that calculated as the corresponding sum of ISDD results for binned sub-populations of agglomerate sizes and densities. Specifically, ignoring polydispersity by using average values for d H and ρ EV introduced a systematic error of ~6%, which is sufficiently negligible to permit a valid prediction of administered dose delivered to cells during a given incubation period. Additional analysis of polydispersity effects is provided in the Supplementary Discussion . Since cellular response to a biologically active substance should relate more closely to the quantity of the substance coming into contact with cells than to its transient initial distribution (for example, administered mass concentration), nanotoxicity in an in vitro system should be better represented in relation to the mean delivered dose based on accurate modelling of mass transport, than to the initial concentration (administered dose) of an ENM. Evaluation of cytotoxicity based on delivered dose calculations, derived from accurate characterization of ENM properties in suspension, may thus help to eliminate the disparity between in vitro and in vivo nanotoxicology outcomes, which in turn could finally enable the kind of efficient and reliable screening methods needed to assess the safety of an ever-increasing number and variety of ENMs being introduced. One important property usually neglected in in vitro nanotoxicology studies is effective density, which determines the fate and transport phenomena and thus the dose delivered to cells in vitro . It also defines the agglomeration state of ENMs in biological media and thus their active surface area. Our findings demonstrate the accuracy and utility of the proposed VCM for estimation of ENM-effective density in suspension and its use in approximating in vitro dosimetry in nanotoxicology. We have shown that effective density estimated by this method can be used to accurately determine the delivered dose of ENM in an in vitro system and that this versatile method may be applied to fractal ENM agglomerates such as metal and metal oxides as well as non-agglomerating nanospheres. It may also be applicable to partially soluble ENMs when supported with time-resolved dissolution characterization in applicable liquid media, although we should note that at present a transport model capable of incorporating such time-variant properties is not available. Our group has also recently successfully utilized the VCM to measure effective density and investigate dosimetry implications for carbon-based ultrafine particles emitted from printing equipment [35] . The primary potential source of error in the VCM approach resides in the use of representative values of the stacking factor, SF . For instance, due to minor differences in polydispersity or agglomerate shape, SF values may not be exactly identical among ENMs of a given class, as we have observed for CeO 2 ( SF =0.61) and SiO 2 ( SF =0.538). Both of these observed values, however, are close to the theoretical value for randomly stacked spheres (0.634), and the corresponding change in ρ EV resulting from such a small deviation from the theoretical SF value is relatively small. Moreover, given the morphological similarity among flame-generated metal oxide ENMs, we believe that differences in SF within this class would generally be small, and that in all cases, the true value of SF would be sufficiently close to the theoretical value that ρ EV could be reliably calculated based on the theoretical value alone. In the context of dosimetry for nanotoxicology, the magnitude of errors in ρ EV and delivered dose resulting from this approximation would be relatively negligible. For several ENMs investigated, the effective density determined by VCM was not greatly different from that calculated using the Sterling equation (although for some ENMs and suspension conditions, the differences were significant). To the best of our knowledge, this is also the first indirect validation of the Sterling equation, which in turn can be employed to correct the standard AUC evaluation with specific respect to the fractal morphology of ENM agglomerates [36] . Although our data suggest that for most metal oxide ENMs the estimation of density using the Sterling equation may be sufficiently accurate, it should be noted that close correspondence between ρ ES and ρ EV was dependent upon a specific choice of DF (2.3), which is slightly larger than the value of 2.1 derived from scattering data and claimed as universally valid for reaction-limited colloidal agglomeration [36] , [37] . Particle characteristics may be influenced by dynamic interactions with proteins commonly found in cell culture media. Any effect of the protein corona will be reflected in the size of the agglomerate and the effective density over the time of the exposure. Thus, the approach described above, of utilizing time-resolved measurements of hydrodynamic diameter and effective density in transport modelling for suspensions that are not stable over time, would also addresses the dynamic nature of the protein corona. Moreover, in addition to our validation experiments discussed above, recent studies have validated the ISDD model for super paramagnetic ion oxide particles and polystyrene beads suspended in protein-supplemented media, suggesting that the dynamic nature of particle–protein interactions likely has little impact on particle transport in vitro [13] , [34] . In conclusion, the simplicity and efficiency of the proposed VCM method will enable nanotoxicologists to incorporate accurate dosimetry modelling in their in vitro system designs, which will be a major step towards the development of inexpensive, accurate and reproducible in vitro screening assays, and a major advancement for nano-environmental health and safety research. Nanomaterials and characterization ENMs investigated are listed in Table 1 . SiO 2 , Fe2O 3 and CeO 2 ENM powders were generated in-house by flame spray pyrolysis using the Harvard Versatile Engineered Nanomaterial Generation System (VENGES) recently developed by the authors [38] , [39] . Additional metal oxide ENM powders were purchased from commercial vendors (SiO 2 and TiO 2 : EVONIK, Essen, Germany; CuO: Sigma-Aldrich, St Louis, MO; ZnO: Alfa Aesar, Ward Hill, MA, USA). Spherical monodisperse gold nanospheres, which were donated by Dr Srinivas Sridhar at Northeastern University, were prepared in suspension as previously described [40] . Briefly, 500 ml of 1 mM HAuCl 4 in a round bottom flask was heated to a rolling boil with vigorous stirring. 50 ml of 38.8 mM sodium citrate solution was added rapidly. After a colour change from pale yellow to purple, indicating formation of gold nanoparticles, boiling was continued for another 15 min, after which the heating source was removed and the solution stirred for an additional 15 min. The solution was filtered through 0.45 μm syringe filters and stored at 4 °C. For powdered ENMs-specific surface area, SSA, defined as the particle surface area per mass (m 2 g −1 ), was determined by the nitrogen adsorption/Brunauer-Emmett-Teller method using a Micrometrics Tristar 3000 (Micrometrics, Norcross, GA, USA) for each ENM. The equivalent primary particle diameter, d BET , was calculated, assuming spherical particles, as where ρ p is the particle density, which was obtained for each particle from the densities of component materials, at 20 °C, reported in the CRC handbook of Chemistry and Physics [41] . Particle crystal size and diameter were also determined by X-ray diffraction using a Scintag XDS2000 powder diffractometer (Scintag, Cupertino, CA, USA), reported here as d XRD . ENM powder primary particle morphology and size were further characterized, and for monodisperse gold nanospheres primary particle diameter was estimated by TEM using a Zeiss Libra 120 microscope (Carl Zeiss GmbH, Jena, Germany). The TEM image of CeO 2 agglomerates suspended in RPMI/10% FBS in Fig. 1 was acquired with a JEOL 2100 microscope (JEOL, Peabody, MA, USA) fitted with a Poseidon 500 electrochemistry liquid cell platform (Protochips, Raleigh, NC, USA). ENM dispersal and characterization in suspension Dispersions were prepared based on a protocol recently developed by the authors [16] . Sonication was performed in deionized water (DI H 2 O) using the critical dispersion sonication energy ( DSE cr ), which was determined as previously described for each ENM [16] . ENMs were dispersed at 5 mg cm −3 in 3 ml of solute in 15 ml conical polyethylene tubes using a Branson Sonifier S-450A (Branson Ultrasonics, Danbury, CT, USA), calibrated by the calorimetric calibration method previously described [16] , [26] , whereby the power delivered to the sample was determined to be 1.75 W, fitted with a 3-inch cup horn (maximum power output of 400 W at 60 Hz, continuous mode, output level 3) in which tubes were immersed so that sample and cup water menisci were aligned. Stock DI H 2 O suspensions were then diluted to final concentrations in either RPMI or F12K cell culture media, each either alone or supplemented with 10% heat inactivated FBS, and vortexed for 30 s. Dispersions were analysed for hydrodynamic diameter ( d H ), polydispersity index, zeta potential ( ζ ) and specific conductance ( σ ) by DLS using a Zetasizer Nano-ZS (Malvern Instruments, Worcestershire, UK). pH was measured using a VWR sympHony pH metre (VWR International, Radnor, PA, USA). Effective density by volumetric centrifugation One millilitre samples of 50,100 or 250 μg cm −3 suspensions of metal oxide ENMs or 1.0 mg cm −3 suspensions of gold nanospheres were dispensed into TPP PCV tubes (Techno Plastic Products, Trasadingen, Switzerland) and centrifuged at 1,000, 2,000 or 3,000 g for 1 h. Agglomerate pellet volumes, V pellet , were measured using a slide rule-like easy-measure device also obtained from the PCV tube manufacturer. Effective agglomerate densities were calculated from V pellet values of triplicate samples for each ENM and condition as described above using equation (4). Media density was calculated from the mass of a 50 ml sample by subtracting the weight of a 50 ml volumetric flask from the weight of the same flask containing 50 ml of media (RPMI or F12K +/− 10% FBS) at 20°C, and agglomerate stacking factors, SF , were determined by AUC as described below. Stacking factor estimation by AUC Dispersions of 0.1 mg cm −3 VENGES CeO 2 ( d BET =5.4 nm) and VENGES SiO 2 ( d BET =18.6 nm) in RPMI+10% FBS, and 0.1 mg cm −3 gold nanospheres ( d H =29 nm) in deionized water were prepared and 400 μl of each were loaded into sample cells of a ProteomeLab XL-A/XL-I An-60 Ti rotor (Beckman Coulter, Brea, CA, USA) equipped with interference optics. Reference cells for CeO 2 , SiO 2 and gold nanospheres were loaded and balanced with either RPMI+10%FBS or deionized water. Samples were centrifuged at 3,000 r.p.m. (122 g ) in a ProteomeLab XL-I analytical ultracentrifuge (Beckman Coulter, Brea, CA, USA). Raw AUC interference data were analysed using Sedfit software, as described elsewhere [19] , [42] , to generate sedimentation coefficient profiles for each sample. The stacking factor, SF , for each ENM was estimated from the weighted mean sedimentation coefficient using equation (6). Effective density estimation by the Sterling model Effective density based on Sterling model [18] was calculated using Supplementary equations (12) and (13) assuming a DF of 2.3. Hydrodynamic diameter, d H , and primary particle diameter, d BET , were measured as described above. In the case of gold nanospheres, which were generated in solution and for which a d BET value therefore does not exist, the primary particle diameter was estimated from TEM images (20 nm). Media density, ρ media , was measured as described above. Inductively coupled plasma mass spectrometry Sample preparation was conducted in a Class 100 trace metal-free clean hood in the Earth and Ocean Sciences Department at Duke University. Samples were agitated for 30 min and vortexed for 1 min prior to preparation. Class A polypropylene test tubes were prewashed in 5% nitric acid bath to remove potential metal contamination. Each sample (0.1 ml) was transferred to the corresponding prelabelled analytical vials and verified gravimetrically to ±0.001 mg. Samples were diluted ~100 × in water purified to 18.2 MΩ cm resistance using a Milli-Q water purification system (Millipore, Bedford, MA, USA), and then acidified using trace metal-free concentrated (15.9 M) Ultrapure nitric acid (Thermo Fisher Scientific, Waltham, MA, USA). Internal standards consisting of known quantities of indium (In) and bismuth (Bi) were added to samples to correct for instrumental drift. All analytical standards, procedural blanks and interference check standards were prepared in an analogous fashion. Cerium content was measured using a Perkin Elmer axial field technology DRC II inductively coupled plasma mass spectrometer (ICP-MS). Prior to sample analysis, the ICP-MS was optimized for sensitivity, stability and to reduce the formation of doubly charged species and oxide interferences using a multi-element tuning solution containing Mg, In, Ba, Ce, Bi and U. Optimization continued until CeO + /Ce + and Ba ++ /Ba + were simultaneously less than 2%. These interferences were quantified to correct for instrumental and procedural backgrounds and isobaric interferences, respectively. During sample analysis, sample lines were rinsed to reduce memory effects by washing sequentially with Milli-Q purified water for 2 min and 2% nitric acid for an additional 2 min between analyses. ICP-MS analyses were conducted as previously reported [43] , [44] . Throughout the analysis, CeO + /Ce + was <2.1%. Ce detection was performed by simultaneously monitoring 140 Ce and 142 Ce. No isobaric interferences were observed for 140 Ce and 142 Ce was corrected for Ne interferences. Calculated solution concentrations obtained from 140 Ce and 142 Ce varied by less than 3.1% on average. [Ce] quantification was obtained using a 7-point external calibration curve spiked with known quantities of Ce in a linear range from 0.050 ng g −1 to 100 ng g −1 (refs 43 , 44 ). Known aliquots of Ce spikes were analysed as unknowns to determine external precision as 2.7%. Five duplicate analyses ( n =5) were performed for all analytes for each sample solution. Delivered dose computation The in vitro sedimentation, diffusion and dosimetry (ISDD) model proposed by Hinderliter et al. [13] was used to calculate the fraction of administered particles deposited standard 96-well plates as a function of time f D ( t ) as previously described [16] . In addition to effective density (estimated either by volumetric centrifugation or from the Sterling model), ISDD model inputs included the hydrodynamic diameter, d H , measured by DLS, the media column height (3.15 mm), temperature (310 K), media density, (1.00 g cm −3 ), media dynamic viscosity (0.00074 Pa s) [13] , and administered (initial suspension) particle concentration (100 μg cm −3 ). For each ENM the model-derived f D ( t ) was fit to a Gompertz sigmoidal equation, where t is time (h), and α is an ENM- and media-specific deposition fraction constant (h −1 ).Solving equation (8) for the time t at which the fraction f D ( t ) of administered particles is delivered yields Equation (9) was used to calculate the time required for delivery of 90% of the administered dose, t 90 , for each ENM dispersion using the specific deposition function constants, α , and an f D ( t ) value of 0.90. Validation of proposed dosimetry methodology ENM powders were irradiated with neutrons for up to 24 h at the Nuclear Reactor Laboratory (Massachusetts Institute of Technology, Cambridge, MA), and the radioactive 141 Ce ENMs (CeO 2 , SiO 2 -coated CeO 2 ) were stored in irradiation tubes. 141 Ce is a gamma emitter with a half-life of 32 days, and the successful production of radioactive ENMs following irradiation was confirmed by gamma energy spectrometry using a Packard gamma counter (Cobra Quantum, Packard Instrument, IL). ENMs were quantified as percentage of total administered mass dose, based on total measured radioactivity (counts per minute, CPM). Concentration calibrations were performed for each ENM by measuring radioactivity for a measured and known total ENM mass in suspension, and measuring radioactivity of serial dilutions by half down to 5 ng cm −3 (data not shown). Hundred microlitres of ENM suspensions at a concentration of 12.5 μg cm −3 was applied to transwell systems without cells for 24 h ( Supplementary Fig. 5 ). Following exposure, all supernatant and transwell inserts were collected from culture plates and set aside for analysis by gamma spectroscopy. Supernatants were collected from the transwell, and transwell inserts were set aside for measurement by gamma spectroscopy. All liquid present in the basolateral compartment of the transwell was then collected, and each basal well was washed three times with PBS and collected. Gamma counts were measured for apical compartments (including supernatant and transwell insert), as well as for the basal compartment (including collected media and PBS wash) by gamma spectroscopy. The mass balance of ENMs measured in the apical and basal compartments was compared with gamma readings for ENM suspensions of equivalent total particle mass (1.25 μg). All experiments were conducted in triplicate. How to cite this article : DeLoid, G. et al. Estimating the effective density of engineered nanomaterials for in vitro dosimetry. Nat. Commun. 5:3514 doi: 10.1038/ncomms4514 (2014). The findings and conclusions in this report are those of the authors and do not necessarily represent the views of the National Institute for Occupational Safety and Health.